Dissociating cognitive and sensory neural plasticity in human superior temporal cortex Disentangling the effects of sensory and cognitive factors on neural reorganization is fundamental for establishing the relationship between plasticity and functional specialization. Auditory deprivation in humans provides a unique insight into this problem, because the origin of the anatomical and functional changes observed in deaf individuals is not only sensory, but also cognitive, owing to the implementation of visual communication strategies such as sign language and speechreading. Here, we describe a functional magnetic resonance imaging study of individuals with different auditory deprivation and sign language experience. We find that sensory and cognitive experience cause plasticity in anatomically and functionally distinguishable substrates. This suggests that after plastic reorganization, cortical regions adapt to process a different type of input signal, but preserve the nature of the computation they perform, both at a sensory and cognitive level. Neural plasticity is the functional and structural reorganization of the brain in response to a given event or set of events. These can arise from physiological or developmental processes, or damage or insult [1] , and can be mediated by cognitive or sensory mechanisms. In congenitally deaf people, neural plasticity has been observed in the superior temporal cortex (STC) [2] , [3] , a region that is associated with auditory and speech sound processing. Although sensory deprivation triggers the reorganization of the cortex, the origin of the anatomical and functional changes observed in the STC of deaf individuals is not only sensory, but also cognitive, as they cannot acquire language through sound, and visual communication strategies, such as the use of sign language and speechreading, need to be developed. Understanding the differential contribution of sensory and cognitive experience to neural reorganization is fundamental for establishing the relationship between plasticity and underlying functional specialization. No dissociation study has been previously undertaken, because it is difficult to characterize the unique contribution of different types of mechanisms in a single model (see ref. 4 ). Instead, previous studies have concentrated on discrete functions. Deafness and sign language provide the ideal model to resolve this. Sign languages have developed naturally in deaf communities. Like spoken languages, they are organized at phonological, morphological, syntactic and semantic levels [5] . Not only do auditory deprivation and language experience mediate plastic changes in deaf individuals, but the robust left-hemisphere involvement in language potentially allows a clear anatomical segregation between them: as the left STC is involved in the processing of language independently of modality (see refs 6 , 7 , 8 ), plastic changes in this region are likely to be mediated by mechanisms supporting the development and acquisition of sign language, and not by general visual processing effects; this constraint may not be true of the right STC. Studying neural reorganization in deaf brains allows us to disentangle plastic changes, and their interaction, both when they are due to life-long sensori-motor adaptation to auditory deprivation, and when they are due to life-long sign language experience. We distinguished between these possibilities by studying the functional magnetic resonance imaging (fMRI) BOLD response to sign-based stimuli in populations of deaf and hearing individuals who were either native signers, or spoken language users without knowledge of sign language. We find that plastic effects in the left STC have a linguistic origin, and are shaped by sign language experience, whereas the right STC also shows plasticity due to sensory deprivation. We conclude that sensory and cognitive factors cause plasticity in anatomically and functionally distinguishable substrates, and that after plastic reorganization, cortical regions preserve the nature of the computation they perform both at a sensory and cognitive level. Plasticity induced by sign language and auditory deprivation We distinguished between these by studying the fMRI BOLD response to sign-based stimuli in two populations of congenitally or early (see Methods) severely to profoundly deaf individuals: (i) ‘Deaf Signers’ (DS): deaf individuals with deaf parents, who were early and proficient (native) users of British Sign Language (BSL), and (ii) ‘Deaf Oral’ (DO): deaf speakers of English, who access language through speechreading and who never learned a sign language. Groups were matched for hearing loss, age and gender. Non-signing hearing native English speakers (Hearing Non-Signers—HN) served as controls. Participants viewed videos of sign-based material (see Methods). This has linguistic content for DS, but only visuo-spatial information for DO and HN. Plastic effects induced by auditory deprivation are expected, independently of linguistic access, in both groups of deaf individuals, but not in the controls. Therefore, we evaluated this effect by comparing each of the deaf groups with the HN group, and then identified commonly activated regions with a conjunction of the comparisons: [DS>HN] and [DO>HN]. In contrast, sign language-induced plasticity should be observed only in DS, who have access to the linguistic content, and not in DO and HN. Thus, this effect was evaluated by comparing the DS group with each of the non-signer groups, with the conjunction of the contrasts: [DS>DO] and [DS>HN]. 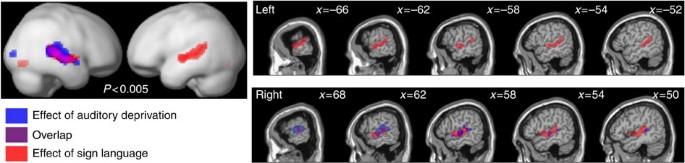Figure 1: Plasticity in the superior temporal cortex induced by sign language and by auditory deprivation. The effect of auditory deprivation was evaluated with the conjunction of T-contrasts [DS>HN] and [DO>HN]; that of sign language with the conjunction [DS>DO] and [DS>HN]. All within a second level analysis of variance for group (N=7) comparison. Results were overlaid on three-dimensional representations of the brain (left) or sagittal slices (right). Images are displayed at a threshold ofP<0.005 (uncorrected) and a spatial threshold of 20 voxels, but activations are discussed only if they reached corrected significance (P<0.05, Family-Wise error (FWE)) at cluster or single voxel level. Coordinates are in Montreal National Institute (MNI) space. Figure 1 shows that differential activations observed in the left STC, in particular in the left superior temporal sulcus, are driven by experience with sign language, and not by auditory deprivation. In the right STC, differential activations are driven both by auditory deprivation and knowing sign language ( Fig. 1 , Table 1 ). These differential activations also occur in anatomically segregated regions, with the effect of auditory deprivation mostly in the lateral portion of the right STC, and the effect of sign language experience extending towards its medial and slightly more anterior part. These differences between the right and left STC are also observed at a lower threshold ( Fig. 2 ), although in this case the effect of deafness is also observed in the posterior part of the middle temporal gyrus and the planum temporale. Figure 1: Plasticity in the superior temporal cortex induced by sign language and by auditory deprivation. The effect of auditory deprivation was evaluated with the conjunction of T-contrasts [DS>HN] and [DO>HN]; that of sign language with the conjunction [DS>DO] and [DS>HN]. All within a second level analysis of variance for group ( N =7) comparison. Results were overlaid on three-dimensional representations of the brain (left) or sagittal slices (right). Images are displayed at a threshold of P <0.005 (uncorrected) and a spatial threshold of 20 voxels, but activations are discussed only if they reached corrected significance ( P <0.05, Family-Wise error (FWE)) at cluster or single voxel level. Coordinates are in Montreal National Institute (MNI) space. Full size image Table 1 Coordinates and descriptive statistics for the effect of sign language and the effect of auditory deprivation. 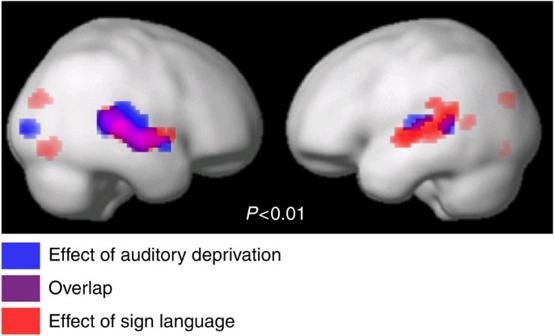Figure 2: Results of plasticity associated with sign language and with auditory deprivation at a lower statistical threshold. The effect of auditory deprivation was evaluated with the conjunction of contrasts [DS>HN] and [DO>HN]; that of sign language with the conjunction of T-contrasts [DS>DO] and [DS>HN]. All within a second-level analysis of variance for group (N=7) comparison. Results were overlaid on three-dimensional representations of the brain (left), and displayed at a threshold ofP<0.01 (uncorrected) and a spatial threshold of 20 voxels. Full size table Figure 2: Results of plasticity associated with sign language and with auditory deprivation at a lower statistical threshold. The effect of auditory deprivation was evaluated with the conjunction of contrasts [DS>HN] and [DO>HN]; that of sign language with the conjunction of T-contrasts [DS>DO] and [DS>HN]. All within a second-level analysis of variance for group ( N =7) comparison. Results were overlaid on three-dimensional representations of the brain (left), and displayed at a threshold of P <0.01 (uncorrected) and a spatial threshold of 20 voxels. Full size image Generalization of results across age and sign languages Two further sets of results show the same pattern of activation and thus confirm and support the generalization of our findings. The first one is from comparisons of larger groups of DS, DO and HN ( Fig. 3 ), in which age was included as a covariate. Deafness was severe/profound in all cases, but because the mean age of the DO group was significantly greater than that of the other two groups, age was used as a covariate in the analysis. The analysis shown in Fig. 3 reveals a pattern of results that is similar to the one obtained when comparing tightly matched groups ( Fig. 1 ). A model that also includes gender as a covariate results in the same pattern of activations. The second set of results is from the comparison of DO and HN to an independent group of deaf native users of a different sign language: ‘Swedish Sign Language Deaf Signers’ (SSL-DS; Fig. 4 ). In agreement with the results presented in Fig. 3 , this analysis shows a pattern of results that is similar to the one obtained when comparing tightly matched groups ( Fig. 1 ). 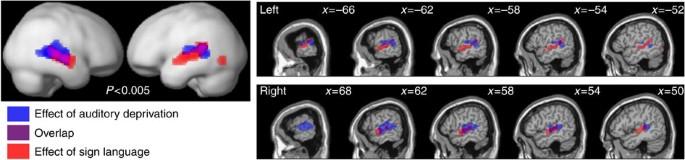Figure 3: Plasticity in the superior temporal cortex induced by sign language and by auditory deprivation with age as a covariate. Results presented in this figure correspond to comparisons between the same three groups described in the main text, but with larger number of participants. Deaf Signers:N=15; Deaf Oral:N=10; Hearing Non-Signers:N=18. Images from each individual were taken to a second level analysis of variance for group comparison. The effect of auditory deprivation was evaluated with the conjunction of T-contrasts [DS>HN] and [DO>HN]; that of sign language with the conjunction [DS>DO] and [DS>HN]. Results were overlaid on three-dimensional representations of the brain (left) or sagittal slices (right). Images are displayed at a threshold ofP<0.005 (uncorrected) and a spatial threshold of 20 voxels, but activations are discussed only if they reached corrected significance (P<0.05, FWE corrected) at cluster or single voxel level. Coordinates are in MNI space. All values±s.e.m. Figure 3: Plasticity in the superior temporal cortex induced by sign language and by auditory deprivation with age as a covariate. Results presented in this figure correspond to comparisons between the same three groups described in the main text, but with larger number of participants. Deaf Signers: N =15; Deaf Oral: N =10; Hearing Non-Signers: N =18. Images from each individual were taken to a second level analysis of variance for group comparison. The effect of auditory deprivation was evaluated with the conjunction of T-contrasts [DS>HN] and [DO>HN]; that of sign language with the conjunction [DS>DO] and [DS>HN]. Results were overlaid on three-dimensional representations of the brain (left) or sagittal slices (right). Images are displayed at a threshold of P <0.005 (uncorrected) and a spatial threshold of 20 voxels, but activations are discussed only if they reached corrected significance ( P <0.05, FWE corrected) at cluster or single voxel level. Coordinates are in MNI space. All values±s.e.m. 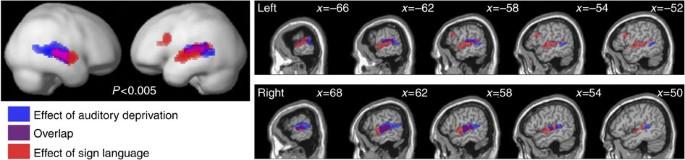Figure 4: Comparison of Deaf Native Swedish Sign Language users and Native English Speakers. Results presented in this figure correspond to comparisons between a group of Deaf Native Swedish Sign Language participants (SSL-DS,N=16), and the groups of Deaf Oral (N=10) and Hearing Non-Signers (N=18) described inFigure 3. Images from each individual were taken to a second level analysis of variance for group comparison. Age was used as a covariate in the analysis. The effect of auditory deprivation was evaluated with the conjunction of T-contrasts [SSL-DS>HN] and [DO>HN]; that of sign language with the conjunction [SSL-DS>DO] and [SSL-DS>HN]. Images are displayed at a threshold ofP<0.005 (uncorrected) and a spatial threshold of 20 voxels, but activations are discussed only if they reached corrected significance (P<0.05, FWE corrected) at cluster or single voxel level. Coordinates are in MNI space. All values±s.e.m. Full size image Figure 4: Comparison of Deaf Native Swedish Sign Language users and Native English Speakers. Results presented in this figure correspond to comparisons between a group of Deaf Native Swedish Sign Language participants (SSL-DS, N =16), and the groups of Deaf Oral ( N =10) and Hearing Non-Signers ( N =18) described in Figure 3 . Images from each individual were taken to a second level analysis of variance for group comparison. Age was used as a covariate in the analysis. The effect of auditory deprivation was evaluated with the conjunction of T-contrasts [SSL-DS>HN] and [DO>HN]; that of sign language with the conjunction [SSL-DS>DO] and [SSL-DS>HN]. Images are displayed at a threshold of P <0.005 (uncorrected) and a spatial threshold of 20 voxels, but activations are discussed only if they reached corrected significance ( P <0.05, FWE corrected) at cluster or single voxel level. Coordinates are in MNI space. All values±s.e.m. Full size image All three different analyses ( Figs 1 , 2 , 3 , 4 ) show the same pattern of effects in the right and left STC. This generalizes our results beyond age, gender and specific characteristics of a particular sign language, pointing towards invariable general plastic reorganization principles. No effect of sign language without explicit linguistic content Furthermore, when participants looked at stimuli with no explicitly linguistic content (cue images consisting of static pictures of handshapes or highlighted parts of the model’s body; see Methods), there was no significant effect of sign language in the whole-brain activation, but the effect of auditory deprivation was preserved ( Fig. 4 ), confirming that the effect observed in the left STC and the anterior and medial part of the right STC in Fig. 1 is driven by linguistic processing. Here, we show that plastic effects in the left STC have a linguistic origin, and are shaped by sign language experience, whereas the right STC also shows plasticity owing to sensory deprivation. More importantly, these results demonstrate that life-long sign language experience and life-long sensori-motor adaptation to auditory deprivation drive plasticity in segregated portions of the cortex. Results in the left STC suggest that, after plastic reorganization, cortical regions can develop their typical function, but adapt to a different type of sensory input, not only to aid perception [9] , [10] , [11] but also for higher-order cognitive functions. Given that auditory stimulation causes activations in the STC in hearing individuals (see ref. 2 for an example), it is clear that in congenitally deaf individuals neural reorganization permits a different type of input to reach these cortices. However, it is less clear if there is also structural or functional reorganization within the region itself. In the left STC, the language-processing function of the region persists and develops as in hearing individuals. Although the function of the right STC has not been as clearly determined, it is possible that this region also preserves its distinct functions, with greater reliance on visual input [12] . To our knowledge, this is the first study that separates the sensory and linguistic components of cross-modal plasticity in two deaf populations with the same sensory loss, but different modalities of language. Previous studies have used stimuli with different levels of linguistic content to look at plasticity in deaf individuals [2] , [3] . However, they have not compared language experiences, typically testing only DS. Even in a case in which the auditory cortex of DS is more responsive to any visual stimulation, this effect could be driven by a top–down mechanism developed with language experience. Another strategy has been to use hearing native signers (hearing children of deaf parents) as controls [8] , [13] , [14] , [15] . With that comparison it is difficult to be conclusive about whether an effect arises from deafness or from different language experience. The development of language in hearing native signers is different from that of deaf native signers [16] , typically involving simultaneous acquisition of signed and spoken language. In our study, sensory experience is constant, demonstrating that left-hemisphere activations observed in the processing of sign language are specifically the result of processing linguistic information, and not an effect of general visual processing. In conclusion, the dissociation shown between the effects in the right and left STC demonstrate that sensory and cognitive factors cause plasticity in anatomically and functionally distinguishable substrates. Furthermore, our findings show that, even after plastic reorganization, cortical regions can preserve the nature of the computation they perform, and only adapt their function to deal with a different input signal, both at a sensory and cognitive level. Participants For our main analysis, presented in Figs 1 and 2 , data were from two groups of seven congenitally or early (before 3 years of age) severely-to-profoundly deaf individuals. These were either DS, who have deaf parents, and are native signers of BSL, or DO, who have hearing parents, and are native speakers of English who access language through speechreading and who have never learned a sign language. A third group of participants with normal hearing who were native speakers of English (HN) were part of a separate control group. Groups were matched for: sensory loss (better-ear pure tone average (PTA; 1, 2, 4 KHz; maximum output of equipment, 100 dB): DS=98.1 dB±3.7 s.e.m. ; DO=94.5 dB±3.3; t [6] =0.64, P =0.54); age (DS=46.3 years±4.4 s.e.m. ; DO=47.3±1; HN=47.6±3.3; t [6] DO,DS =0.23, P =0.82; t [6] DO,HG =0.09, P =0.93; t [6] HG,DS =0.2, P =0.81); and gender (three male and four female in each group). All deaf participants learned their preferred language from infancy. Participants in the DS group were native signers of BSL (at least one deaf parent), and on average (data obtained from 6/7 participants owing to experimental time constraints), they indicated their level of proficiency of BSL to be 6.17 on a scale of 1–7 (1=not very good at all; 7=excellent). All DS communicated with the researchers in BSL. The DO group had on average adult reading skills (35.6 points±1.19 s.e.m. ), as measured with the revised Vernon–Warden Reading Comprehension Test [17] , ranging from 32–38 (data obtained from 6/7 participants owing to experimental time constraints). All DO participants communicated with the researchers in English. Participants in the DS and HN groups were recruited from local databases. Most of the participants in the DO group were recruited through an association of former students of a local oral-education school. Because of changing attitudes towards sign language, even deaf people raised in a completely oral environment and who developed a spoken language successfully are now more likely to be interested in learning to sign as young adults. Sign language knowledge was an exclusion criterion for the DO group. For this reason, all the participants in the DO group were more than 40 years of age, and participants in the other two groups were chosen to match them. Results presented in Fig. 3 correspond to comparisons between the same three groups described above, but with larger number of participants. DS: N =15; age=38.37±3.22 years; gender=6 male, 9 female; PTA=98.2±2.4 dB; DO: N =10; age=49.8±1.7; gender=6 male, 4 female; PTA=95.2±2.6; HN: N =18; age=37.55±2.3; gender=9 male, 9 female. Results described in Fig. 4 also include a group of Deaf Native Swedish Sign Language users ((SSL-DS): N =16; age=33.25±2.4 years; gender=6 male, 10 female; PTA=99.6±2.6 dB). Participants in the group of Deaf Native Swedish Sign Language users were recruited from local Deaf groups in Sweden. Their preferred language was Swedish Sign Language, and this was also the language they used to communicate with the researchers. All SSL-DS participants had at least one deaf parent. Participants travelled to Birkbeck-UCL Centre of Neuroimaging in London to take part in the study (the aims of which include a cross-linguistic comparison that will be reported elsewhere). All participants were compensated for their travel and accommodation expenses. All participants gave written consent to take part in the study, and all procedures followed the standards set by the Declaration of Helsinki, and were approved by the local ethics committee. Experimental design Results presented in this paper are part of a larger study investigating cross-lingual differences in sign language processing, which will be reported in separate papers. Stimuli consisted of videos of sign-based material, each one of 2–3 s of duration. There were four types of signs: (a) BSL; (b) Swedish Sign Language; (c) Cognates (signs shared by both languages owing to their iconic nature); and (d) Non-signs. Non-signs were either reported by or created following the procedures described in Orfanidou et.al . [18] There were four scanning runs, each consisting of 3 blocks of 12 videos per condition (12 blocks per run), with an inter-trial interval of 4.5 s on average. A baseline period of 15 s, consisting of the image of the model without making any movement with his hands, appeared between blocks. Participants’ task was to indicate with a button-press if the sign presented in each video had the same hand-shape or same location as a cue presented just before the onset of the block. The cues consisted of static pictures of handshapes or highlighted parts of the model’s body. The task could be performed by anyone independently of sign language knowledge but may tap phonological knowledge of sign language (there were no significant differences in performance across groups). 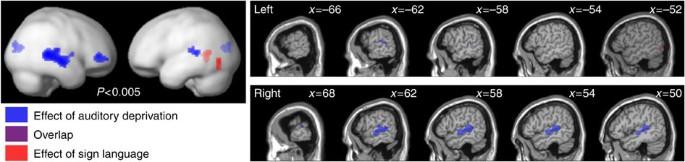Figure 5: Stimuli with no linguistic content reveal only plastic changes induced by auditory deprivation. The figure shows the results obtained when comparing the activations elicited by the Cue images displayed just before the sign-based material. Cue images consisted of static pictures of handshapes or highlighted parts of the model’s body, and they did not have explicit linguistic content. Results presented in this figure correspond to comparisons between the three tightly matched groups of Deaf Signers (N=7), Deaf Oral (N=7) and Hearing Non-Signers (N=7; all as inFig. 1). Within a second level analysis of variance for group comparison, the effect of auditory deprivation was evaluated with the conjunction of T-contrasts [DS>HN] and [DO>HN]; that of sign language with the conjunction [DS>DO] and [DS>HN]. All results were overlaid on three-dimensional representations of the brain (left) or sagittal slices (right). Images are displayed at a threshold ofP<0.005 (uncorrected) and a spatial threshold of 20 voxels, but activations are discussed only if they reached corrected significance (P<0.05, FWE) at cluster or single voxel level. Only the cluster in the right superior temporal cortex reaches significance atP<0.05 (FWE corrected). Coordinates are in MNI space. Figure 5: Stimuli with no linguistic content reveal only plastic changes induced by auditory deprivation. The figure shows the results obtained when comparing the activations elicited by the Cue images displayed just before the sign-based material. Cue images consisted of static pictures of handshapes or highlighted parts of the model’s body, and they did not have explicit linguistic content. Results presented in this figure correspond to comparisons between the three tightly matched groups of Deaf Signers ( N =7), Deaf Oral ( N =7) and Hearing Non-Signers ( N =7; all as in Fig. 1 ). Within a second level analysis of variance for group comparison, the effect of auditory deprivation was evaluated with the conjunction of T-contrasts [DS>HN] and [DO>HN]; that of sign language with the conjunction [DS>DO] and [DS>HN]. All results were overlaid on three-dimensional representations of the brain (left) or sagittal slices (right). Images are displayed at a threshold of P <0.005 (uncorrected) and a spatial threshold of 20 voxels, but activations are discussed only if they reached corrected significance ( P <0.05, FWE) at cluster or single voxel level. Only the cluster in the right superior temporal cortex reaches significance at P <0.05 (FWE corrected). Coordinates are in MNI space. Full size image Data collection and analysis Functional gradient-echo EPI images (repetition time (TR)=2975, ms, TE=50 ms, field of view (FOV) FOV=192 × 192 mm, voxel size=3 mm 3 , 35 slices) were acquired on a Siemens Avanto 1.5T scanner equipped with a 32-channel head coil. The first seven volumes of each run were discarded to allow for T1 equilibration effects. Data were analysed using Matlab 7.10 (Mathworks Inc., MA, USA) and SPM8 (Wellcome Trust Centre for Neuroimaging, London, UK). Images were realigned, coregistered, normalized and smoothed (8 mm FWHM Gaussian kernel) following SPM8 standard pre-processing procedures. Anatomical images were collected using magnetization-prepared rapid acquisition with gradient echo (TR=2730, ms, echo time (TE)=3.57 ms, voxel size=1 mm 3 , 176 slices). Analysis was conducted by fitting a general linear model (GLM) with regressors representing each stimulus category, task, baseline and cue periods. For every regressor, events were modelled as a boxcar of the adequate duration, convolved with SPM’s canonical haemodynamic response function and entered into a multiple regression analysis to generate parameter estimates for each regressor at every voxel. Movement parameters were derived from the realignment of the images and included in the model as regressors of no interest. Contrasts for each experimental condition ([Condition>Baseline]) were defined individually for each participant, and taken to a second level analysis of variance for group comparison, collapsing across conditions. How to cite this article: Cardin.V et al. Dissociating cognitive and sensory neural plasticity in human superior temporal cortex. Nat. Commun. 4:1473 doi: 10.1038/ncomms2463 (2013).